G1-arrested newborn cells are the predominant infectious form of the pathogenBrucella abortus Several intracellular pathogens, such as Brucella abortus , display a biphasic infection process starting with a non-proliferative stage of unclear nature. Here, we study the cell cycle of B. abortus at the single-cell level, in culture and during infection of HeLa cells and macrophages. The localization of segregation and replication loci of the two bacterial chromosomes indicates that, immediately after being engulfed by host-cell endocytic vacuoles, most bacterial cells are newborn. These bacterial cells do not initiate DNA replication for the next 4 to 6 h, indicating a G1 arrest. Moreover, growth is completely stopped during that time, reflecting a global cell cycle block. Growth and DNA replication resume later, although bacteria still reside within endosomal-like compartments. We hypothesize that the predominance of G1-arrested bacteria in the infectious population, and the bacterial cell cycle arrest following internalization, may constitute a widespread strategy among intracellular pathogens to colonize new proliferation niches. Several pathogenic bacteria such as Legionella , Salmonella , Chlamydia, Francisella and Brucella replicate inside mammalian host cells. These species all display a biphasic infectious mode in which the increase of the intracellular bacterial population occurs only after a relatively long non-proliferative period characterized by a very low number of bacteria per cell [1] . The presence of this first non-proliferative phase suggests that the cell cycle progression of these pathogens could be stalled during this step. However, despite its likely importance for the success of the infection, the cell cycle progression of intracellular pathogens has never been investigated so far. In addition, whether individual bacterial cells keep increasing their size during the non-proliferative phase is unknown. The facultative intracellular pathogen Brucella abortus is an alphaproteobacterium causing brucellosis, a worldwide zoonosis [2] . B. abortus infection occurs in two clear successive steps in the HeLa cellular model of infection. The first step of infection, in which bacteria transit within endocytic vacuoles carrying the lysosomal membrane-associated protein-1 (Lamp-1) marker, is characterized by a stable number of colony-forming units (CFU) [3] . A similar non-proliferative stage is also observed for B. abortus during infection of professional phagocytes such as macrophages [4] . During the second step of infection, the bacteria are found in endoplasmic reticulum (ER)-like compartments where the number of CFU strongly increases suggesting an uninterrupted bacterial cell cycle at this stage [4] , [5] , [6] . Regarding its cell cycle, B. abortus shares features with Caulobacter crescentus , an aquatic alphaproteobacterium used as a model for the study of bacterial development [7] . Indeed, both bacterial species display a common master cell cycle regulator and divide asymmetrically [8] , [9] , [10] . Nevertheless, C. crescentus and B. abortus harbour very different lifestyles. In sharp contrast to C. crescentus , B. abortus cell cycle features original traits for which the mechanisms remained uninvestigated. Indeed, B. abortus displays an atypical unipolar growth mode as well as a particular genomic content composed of two replicons bearing specific partitioning systems [11] , [12] . On the one hand, the unipolar mode of growth was highlighted by the labelling of bacteria with Texas red conjugated to succinimidyl ester (TRSE) that allows, after growth resumption, the visualization of an unlabelled pole and subsequently unlabelled or partially labelled daughter cells [12] . On the other hand, the B. abortus genome is distributed in two replicons of unequal sizes, a large chromosome (chrI; 2.1 Mb) and a small chromosome (chrII; 1.2 Mb) [13] . In fact, although partially described for two other alphaproteobacteria [14] , the multipartite genome replication and segregation have been poorly investigated in this group. B. abortus chrI encodes a predicted ParAB segregation system containing the centromere-like parS site [15] as in C. crescentus and a replication origin ( oriI ) also located close to hemE gene [8] , [16] . ChrII belongs to the alphaproteobacterial chromids, that is, replicons sharing chromosomic and plasmidic features, which carry a repABC cassette [17] . The repABC operon encodes two trans -acting proteins, RepA and RepB, suggested to be involved in the segregation of the chromids and the centromere-binding sequence repS that is recognized by RepB [15] , [18] , whereas the gene coding for the chromid replication initiator repC is predicted to house the replication origin ( oriII ) [18] . Despite the presence of a repABC cassette on the majority of chromids in alphaproteobacteria, none of its components has been localized in living cells so far. The visualization of bacterial cell growth by TRSE labelling [12] and of the chromosomal replication status by the number of origin regions should in principle allow the distinction of three successive stages during the cell cycle of B. abortus : (i) a ‘newborn’ (Nb) stage composed of bacteria that have not yet initiated the replication of one of their replicons; (ii) an ‘intermediate’ (Int) stage where growing bacteria replicate their genome without detectable division; (iii) a last stage composed of ‘predivisional’ (Pd) bacteria, that is, those displaying a constricting division site. At the chromosomal replication level, the Nb stage corresponds thus to the G1 phase of the cell cycle, while the Int and Pd types that replicate their genome correspond to the S and G2 phases. Here, we report the characterization of the genome replication of B. abortus for both chromosomes during in vitro culture as well as under infection conditions. We find that the chromosomes are oriented along the cell length axis and that oriII is duplicated after oriI , suggesting a spatio-temporal organization of the multipartite genome. Importantly, our segregation markers also show that a high proportion of intracellular B. abortus are found in G1 at the entry and remain blocked at that particular stage during an extended period of the non-proliferative phase of the infection, in HeLa cells and in macrophages. In addition, we show that these bacteria are also arrested for growth during this step. Both observations indicate that the B. abortus newborn cell type is the predominant infectious form. Surprisingly, we observe in HeLa cells that the cell cycle already resumes in compartments labelled with the endosomal Lamp-1 marker. The bacterial cell cycle is thus coordinated with the invasion and the trafficking of the bacterium in the host cells. The oriI localizes at one or both bacterial cell poles We investigated the localization pattern of the putative centromere-binding protein ParB in B. abortus as a reporter of the chrI replication status. We assumed that ParB binds to parS in B. abortus since, when ectopically produced in E. coli , a B. abortus YFP–ParB fusion formed foci in the presence of its predicted centromere-like parS sequences ( Supplementary Fig. 1a ), as demonstrated for other ParB/ parS complexes [19] , [20] . In B. abortus , we thus generated a strain allowing the localization of ParB through the replacement of the parB open reading frame by an mcherry-parB fusion. This strain displayed morphological defects that were alleviated by the addition of an intact copy of parB ( Supplementary Fig. 2a–d,f ). The resulting merodiploid mcherry-parB strain strictly displayed one or two mCherry-ParB foci and a wild-type genomic content as indicated by flow cytometry ( Supplementary Fig. 2d ). We observed that 26% of bacteria featured one focus and 74% of bacteria contained two foci of mCherry-ParB ( n =4,846 cells in a representative experiment) during in vitro culture meaning that 26% of the bacterial population did not initiate replication of chrI. Smaller cells, corresponding to the newly generated bacteria (newborns), were characterized by the presence of only one mCherry-ParB focus ( Supplementary Fig. 2c,e ). Moreover, this unique focus was closely associated to the old pole as it localized opposite to a new pole marker, IfoP-YFP ( Fig. 1a , Supplementary Fig. 3a,b ), identified in genome-wide screen for polar proteins in B. abortus (see Supplementary Fig. 4a–f and Supplementary Note 1 ) [21] . Each bacterial cell is characterized by a new pole and an old pole [22] , the new poles are generated by cell division, and the new pole becomes an old pole when the next cell division is completed. In a few larger bacteria, two close mCherry-ParB foci were observed at the old pole, while in the rest of the larger cells, these foci were strictly found at opposite poles. These observations suggest a mechanism of segregation similar to the C. crescentus chromosome, in which the old-pole-associated ParB bound to parS sequences duplicates when replication starts and one of the parS /ParB complexes then migrates to the opposite pole during segregation [23] . 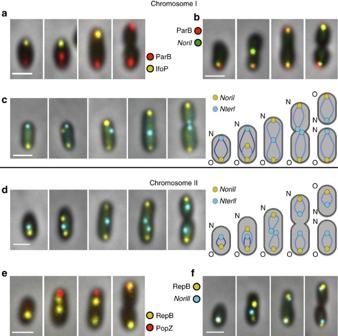Figure 1: Localization patterns of segregation markers and specific genomic regions of bothB. abortuschromosomes. (a) Representative cells producing mCherry-ParB (red) and IfoP-YFP (yellow, new pole marker, seeSupplementary Fig. 4). The second picture shows a probable recent event of ParB duplication. (b) Colocalization between mCherry-ParB (red) andNoriI-targeted YFP (green) in representative cells. (c) TypicalNoriI-targeted YFP (yellow) andNterI-targeted CFP (blue) localization patterns and schematic representation of chrI orientation along the bacterial cell cycle. PolarNterIregion was never found when duplicatedNoriIis bipolar. O represents the old pole and N the new pole locations. (d) TypicalNoriII-targeted YFP (yellow) andNterII-targeted CFP (blue) localization patterns and schematic representation of chrII orientation along the bacterial cell cycle. (e) Representative cells producing YFP-RepB (yellow) and PopZ-mCherry (red) fusions (PopZ-mCherry is a new pole marker, seeSupplementary Fig. 7). (f) Partial colocalization between YFP-RepB (yellow) andNoriII-targeted CFP (blue). Larger fields of the different localization patterns are available inSupplementary Fig. 3afor mCherry-ParB and IfoP-YFP, inSupplementary Fig. 3dfor mCherry-ParB andNoriI-targeted YFP, inSupplementary Fig. 6aforNoriII-YFP andNterII-CFP, inSupplementary Fig. 6dfor YFP-RepB andNoriII-CFP. Scale bars, 1 μm. Figure 1: Localization patterns of segregation markers and specific genomic regions of both B. abortus chromosomes. ( a ) Representative cells producing mCherry-ParB (red) and IfoP-YFP (yellow, new pole marker, see Supplementary Fig. 4 ). The second picture shows a probable recent event of ParB duplication. ( b ) Colocalization between mCherry-ParB (red) and NoriI -targeted YFP (green) in representative cells. ( c ) Typical NoriI -targeted YFP (yellow) and NterI -targeted CFP (blue) localization patterns and schematic representation of chrI orientation along the bacterial cell cycle. Polar NterI region was never found when duplicated NoriI is bipolar. O represents the old pole and N the new pole locations. ( d ) Typical NoriII -targeted YFP (yellow) and NterII -targeted CFP (blue) localization patterns and schematic representation of chrII orientation along the bacterial cell cycle. ( e ) Representative cells producing YFP-RepB (yellow) and PopZ-mCherry (red) fusions (PopZ-mCherry is a new pole marker, see Supplementary Fig. 7 ). ( f ) Partial colocalization between YFP-RepB (yellow) and NoriII -targeted CFP (blue). Larger fields of the different localization patterns are available in Supplementary Fig. 3a for mCherry-ParB and IfoP-YFP, in Supplementary Fig. 3d for mCherry-ParB and NoriI -targeted YFP, in Supplementary Fig. 6a for NoriII -YFP and NterII -CFP, in Supplementary Fig. 6d for YFP-RepB and NoriII -CFP. Scale bars, 1 μm. Full size image To confirm the localization of the mCherry-ParB fusion in B. abortus , we used two exogenous parS /ParB systems derived from exogenous plasmids for the localization of genomic regions of interest ( parS pMT1 or parS P1 being bound by YFP-ParB pMT1 or CFP-ParB P1 , respectively) [24] , [25] . A parS pMT1 sequence was inserted in a region neighbouring oriI (termed NoriI ). The NoriI region labelled by YFP-ParB pMT1 localized close to the old-pole marker PdhS-mCherry [26] or with the single focus mCherry-ParB at the old pole ( Fig. 1b , c , Supplementary Figs 2f and 3c ). Co-labelling experiments showed that 92% of the cells simultaneously displayed either one or two foci of both mCherry-ParB and YFP-labelled NoriI ( n =1,378 cells in a representative experiment; Fig. 1b and Supplementary Fig. 3d ). Together with the localization data, the correlation between the numbers of mCherry-ParB ( oriI ) and NoriI foci validate the use of mCherry-ParB as a reporter for the replication initiation and segregation of chrI origin. Thus, smaller cells harbouring only one mCherry-ParB focus found in minority in liquid culture correspond to bacteria in which chrI replication has not been initiated. The oriII is not fixed within B. abortus cells We investigated the replication of chrII by constructing a B. abortus strain expressing yfp-repB from its chromosomal locus. Similar to ParB and parS , the spatial distribution of YFP-RepB was affected by the presence of its cognate repS sequence from Brucella oriII when ectopically produced in E. coli ( Supplementary Fig. 1b ). In B. abortus , we observed that the yfp-repB cell population displayed a genomic content and morphology comparable to the wild-type strain ( Supplementary Fig. 5a,d ). YFP-RepB formed either one or two clear foci per bacterium (in 49% or 51% of the population, respectively, n =7,127 bacteria in a representative experiment) ( Supplementary Fig. 5a ). The bacteria displaying only one focus were smaller than those displaying two foci ( Supplementary Fig. 5b ). In these cells, the unique RepB focus was found at various positions between the old pole and midcell ( Fig. 1e ) and did not colocalize with the new pole marker PopZ-mCherry ( Supplementary Figs 6a,b and 7a–c ). In bacteria containing two YFP-RepB foci, the distribution pattern of the fusion does not adopt a defined position at the ¼ and ¾ cell positions, as it is the case for some plasmids or chrII of V. cholerae [27] ( Fig. 2b ). In late predivisional cells, two YFP-RepB foci were distributed closer to the poles. Time-lapse experiments showed that a single focus of YFP-RepB is moving in the smaller cells and duplicates in a region ranking between the old pole and midcell. On duplication, the distance between mobile YFP-RepB foci was increasing concomitantly with cell growth, suggesting that the duplicated oriII regions are progressively moving apart ( Supplementary Fig. 5c and Supplementary Movie 1 ). Similarly to our previous experiment with chrI, we inserted a parS P1 sequence 18 kb away from oriII (in a region named NoriII ) in the yfp-repB strain ( Supplementary Fig. 5e ). Colocalization experiments showed that 82% of the cells displayed the same number of foci between YFP-RepB and CFP-labelled NoriII ( n =3,447 bacteria in a representative experiment; Fig. 1f and Supplementary Fig. 6d,e ). These results therefore validate YFP-RepB as a reliable marker of the replication and segregation of chrII origin since the majority of bacteria containing a single YFP-RepB ( oriII ) focus contain only one copy of NoriII . 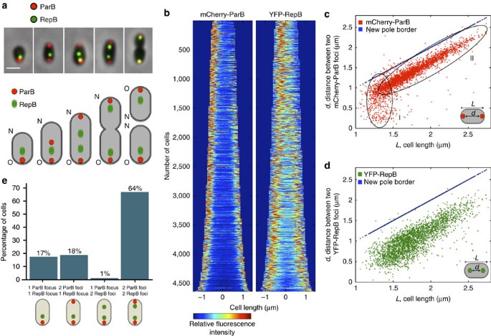Figure 2: Distinct localization patterns of the two replication origins and systematic delay of replication initiation of chrII. (a) Typical localization patterns of cells producing mCherry-ParB (red) and YFP-RepB (green) fusions and schematic representation of their positions. Fuzzy green dots represent the intracellular mobility of YFP-RepB. A larger field of view is available atSupplementary Fig. 9c. O represents the old pole and N the new pole locations. Scale bar, 1 μm. (b) Demographic representation of mCherry-ParB and YFP-RepB fusions (n=4,636 cells). Cells are sorted according to their length (small cells are on the top), and in each cell the fluorescence intensity of mCherry-ParB or YFP-RepB is represented by a colour code, the low intensity corresponding to dark blue, while high intensity is shown in red (c–f) Representation of the distance between two mCherry-ParB or two YFP-RepB foci according to the cell length. (c) Distance between two mCherry-ParB foci can be classified in two specific classes (I and II) suggesting a two-step segregation mechanism. (d) Distance between two YFP-RepB foci display a single progressive separation process. (e) Proportion of cells for different numbers of mCherry-ParB (red) and YFP-RepB (yellow) spots (n=4,636 cells). Almost no bacteria displaying two RepB foci but only one ParB spot were detected suggesting that replication initiation of chrI origin occurs before replication of chrII. Figure 2: Distinct localization patterns of the two replication origins and systematic delay of replication initiation of chrII. ( a ) Typical localization patterns of cells producing mCherry-ParB (red) and YFP-RepB (green) fusions and schematic representation of their positions. Fuzzy green dots represent the intracellular mobility of YFP-RepB. A larger field of view is available at Supplementary Fig. 9c . O represents the old pole and N the new pole locations. Scale bar, 1 μm. ( b ) Demographic representation of mCherry-ParB and YFP-RepB fusions ( n =4,636 cells). Cells are sorted according to their length (small cells are on the top), and in each cell the fluorescence intensity of mCherry-ParB or YFP-RepB is represented by a colour code, the low intensity corresponding to dark blue, while high intensity is shown in red ( c – f ) Representation of the distance between two mCherry-ParB or two YFP-RepB foci according to the cell length. ( c ) Distance between two mCherry-ParB foci can be classified in two specific classes (I and II) suggesting a two-step segregation mechanism. ( d ) Distance between two YFP-RepB foci display a single progressive separation process. ( e ) Proportion of cells for different numbers of mCherry-ParB (red) and YFP-RepB (yellow) spots ( n =4,636 cells). Almost no bacteria displaying two RepB foci but only one ParB spot were detected suggesting that replication initiation of chrI origin occurs before replication of chrII. Full size image Both chromosomes are oriented along the cell length The localization patterns of both replication origins suggest that the two chromosomes display a defined spatial organization in B. abortus . Consistent with this idea, a strain simultaneously labelled at NoriI and at a region neighbouring the terminator of chrI ( NterI ) showed that NterI is located at the new pole when cells displayed a single old-pole-associated NoriI ( Fig. 1c and Supplementary Fig. 3c ). This is reminiscent of the orientation of the single chromosome in C. crescentus [28] . In dividing cells, NterI was detected as a single focus or sometimes as two close foci near the constriction site while NoriI strictly occupied both poles ( Fig. 1c ), also consistent with the positions of the chromosomal origin and terminator into dividing C. crescentus cells. We also monitored the orientation of chrII by colocalizing NoriII with a region neighbouring terII ( NterII ) ( Supplementary Fig. 5e ). Although chrII is oriented along the cell length axis similar to chrI, we found that NoriII is less tightly associated to the poles than NoriI and that NterII is commonly found close to midcell ( Fig. 1d and Supplementary Fig. 6c ). Moreover, NterII is often seen duplicated even in bacteria that do not exhibit a detectable constriction, suggesting that the separation of the chrII sister copies occurs before the segregation of duplicated terI regions, similarly to V. cholerae [29] ( Fig. 1d ). Consistent with this observation, 25% of the cells displayed one focus of NterI and two foci of NterII , while less than 1% of the cells displayed two NterI and one NterII foci ( n =1,305 cells in a representative experiment) in a strain in which both terminator regions were labelled ( Supplementary Fig. 8a ). Hence, the two chromosomes of B. abortus display a distinct spatial organization within the cell. The replication of chrI is initiated first Because B. abortus genome is distributed on two chromosomes, the G1-to-S phase transition could occur either by initiation of chrI replication (visualized by duplication of oriI ) or by replication initiation of chrII (duplication of oriII ), or both. To test this, we constructed a strain producing both mCherry-ParB and YFP-RepB fusions used as markers of oriI and oriII , respectively ( Fig. 2a and Supplementary Fig. 9a–d ). Demographic representations confirmed our data showing that both non-duplicated origins occupy the old pole region although the origin of chrII appears not as closely associated with the pole as the origin of chrI ( Fig. 2b ). Next, we measured the distance between the two mCherry-ParB foci and the two YFP-RepB foci, when both duplicated fusions were detectable. Two classes of bacteria (I and II) could be distinguished from the distance between two mCherry-ParB foci plotted as a function of the cell length (used here as a reporter of cell cycle progression), suggesting that the segregation process can be separated in at least two steps ( Fig. 2c ). Considering the old-pole mCherry-ParB spot as the first focus, class I included the smaller intermediate bacteria in which the second mCherry-ParB focus was either found in the cell body or already at the new pole, which is consistent with a rapid migration process. For cells of class II, the distance between the two mCherry-ParB foci increased similarly to the distance separating the two poles of the growing bacterium. In contrast, the separation of the duplicated YFP-RepB foci seemed to happen in a single step. These data show that the ParAB- and RepAB-based modes of origin segregation follow distinct dynamics ( Fig. 2d ). Strikingly, when comparing the number of foci for both fusions, we found that 18% of the population possess two mCherry-ParB foci but only one YFP-RepB focus, while very few cells (0.9%) displayed one mCherry-ParB focus and two YFP-RepB foci ( n =4,636 cells in a representative experiment; Fig. 2e ). This indicates that the replication of chrI is initiated before the replication of chrII. The observation of a double NoriI NoriII -labelled strain was consistent with this conclusion ( Supplementary Fig. 8b ). Indeed, we found 13% of cells displaying two NoriI foci but only one NoriII focus while the opposite distribution was only found in 2% of the bacteria ( n =706 cells in a representative experiment). In addition, YFP-RepB was duplicated only in bacteria displaying a strict bipolar mCherry-ParB localization suggesting that the replication initiation of oriII is coordinated with the replication initiation and/or segregation of oriI in B. abortus ( Supplementary Fig. 9e,f ). Invasive bacteria are mainly in G1 phase Since a typical cellular infection is characterized by a first non-proliferative stage, we investigated the progression of B. abortus cell cycle at this step and compared it with the proliferative phase. We therefore took advantage of ParB and RepB fusions as reliable markers of the initiation of replication of both chromosomes for single bacterial cell analysis in host cells. HeLa cell infections were performed with the merodiploid mcherry-parB strain producing diffuse GFP ( mcherry-parB GFP strain) or with the yfp-repB strain. Infected cells were observed at 6 h (before the end of the non-proliferative phase) and at 18 h (proliferative phase) post infection (PI; Fig. 3 ). During the proliferative stage, the localization patterns of mCherry-ParB and YFP-RepB were similar to those observed during in vitro cultures. However, during the non-proliferative stage of the infection (6 h PI), the population distribution showed a drastic bias towards the newborn cell type. Indeed, 79±2% ( n =313 of total bacteria, 2% being the s.d.) of mcherry-parB GFP bacteria displayed a unipolar mCherry-ParB focus, while the proportion of bacteria with only one focus was 26% ( n =4,846 cells in a representative experiment) and 35±0.5% ( n =550 of total bacteria) during in vitro cultures and proliferative stage, respectively ( Fig. 3a,b,f ). Incubation of B. abortus with HeLa cell culture medium did not result in a strong enrichment at the G1 stage of the cell cycle since 36% of the bacteria display one focus of mCherry-ParB ( n =821 of total bacteria). Regarding chrII, 85±2.5% ( n =576 of total bacteria) of bacteria displayed only one YFP-RepB focus compared with 49% ( n =7,127 bacteria in a representative experiment) during in vitro cultures and 48±0.8% ( n =459 of total bacteria) at 18 h PI ( Fig. 3c,d,f ). These data strongly suggest that the majority of the bacteria remain in the G1 phase during the non-proliferative stage of the infection. This predominant bacterial G1 phase was further confirmed by using the double NoriI NoriII -labelled strain. Consistent with the ParB and RepB results, we observed that 80±4.7% ( n =400 of total bacteria) of the bacteria exhibited only one focus of labelled NoriI and NoriII regions at 6 h PI, corresponding to the cells that contain only one copy of each chromosome ( Fig. 3e,f ). 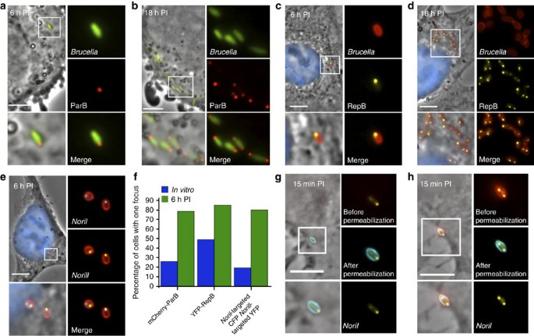Figure 3: Single foci of mCherry-ParB, YFP-RepB, CFP-labelledNoriIand YFP-labelledNoriIIfusions are predominant at 6 h PI. (a,b) Bacteria producing mCherry-ParB (red) fusion and diffuse GFP (green) at (a) 6 h and (b) 18 h PI. At 6 h PI, most bacteria showed (79%) one mCherry-ParB focus. (c,d)B. abortus(red) producing YFP-RepB (yellow) fusion at 6 h (c) and 18 h (d) PI respectively. At 6 h PI, most bacteria showed (85%) one YFP-RepB focus. (e)B. abortus(red) with CFP-labelledNoriI(cyan) and YFP-labelledNoriII(yellow) at 6 h PI. Most bacteria showed (80%) one focus for both fusions. Inctoe, nuclei are stained with 4',6-diamidino-2-phenylindole (blue). (f) Comparison of the percentage of cells displaying one fluorescent focus for mCherry-ParB, YFP-RepB, CFP-labelledNoriIand YFP-labelledNoriIIrespectivelyin vitro(grey) and 6 h PI (black) conditions. (g,h)B. abortusYFP-labelledNoriIat 15 min PI after performing a dual labelling. Intracellular bacteria (g) are not labelled with antibodies used before permeabilization (red), while extracellular bacteria (h) are recognized by antibodies used before and after permeabilization (red and cyan, respectively). One or two intracellular bacteria were found in each infected cell, and most of these bacteria displayed only one focus of YFP-labelledNoriI(73%). Scale bars, 5 μm. Figure 3: Single foci of mCherry-ParB, YFP-RepB, CFP-labelled NoriI and YFP-labelled NoriII fusions are predominant at 6 h PI. ( a , b ) Bacteria producing mCherry-ParB (red) fusion and diffuse GFP (green) at ( a ) 6 h and ( b ) 18 h PI. At 6 h PI, most bacteria showed (79%) one mCherry-ParB focus. ( c , d ) B. abortus (red) producing YFP-RepB (yellow) fusion at 6 h ( c ) and 18 h ( d ) PI respectively. At 6 h PI, most bacteria showed (85%) one YFP-RepB focus. ( e ) B. abortus (red) with CFP-labelled NoriI (cyan) and YFP-labelled NoriII (yellow) at 6 h PI. Most bacteria showed (80%) one focus for both fusions. In c to e , nuclei are stained with 4',6-diamidino-2-phenylindole (blue). ( f ) Comparison of the percentage of cells displaying one fluorescent focus for mCherry-ParB, YFP-RepB, CFP-labelled NoriI and YFP-labelled NoriII respectively in vitro (grey) and 6 h PI (black) conditions. ( g , h ) B. abortus YFP-labelled NoriI at 15 min PI after performing a dual labelling. Intracellular bacteria ( g ) are not labelled with antibodies used before permeabilization (red), while extracellular bacteria ( h ) are recognized by antibodies used before and after permeabilization (red and cyan, respectively). One or two intracellular bacteria were found in each infected cell, and most of these bacteria displayed only one focus of YFP-labelled NoriI (73%). Scale bars, 5 μm. Full size image Collectively, our results show that the majority of B. abortus cells are blocked in the G1 phase after 6 h in the non-proliferative step of the HeLa cell infections. Because the G1 status is characteristic of the newborn cells, which did not resume cell cycle progression since cell division, and because most bacteria did not grow intracellularly until 6 h PI (see below), these results strongly suggest that the newborns have preferentially invaded the host cells. To confirm this, we observed B. abortus NoriI region labelled by YFP-ParB pMT1 at 15 min PI, that is, just after the entry. Intracellular bacteria were discriminated from extracellular bacteria using a double immunolabeling, before or after permeabilization of the infected cells. Only one or two intracellular bacteria were observed per host cell, and these intracellular bacteria most frequently displayed only one focus of NoriI region (73±3%, n =309 of total bacteria) demonstrating that the newborns constitute the predominant invasive form of B. abortus ( Fig. 3g,h ). Bacterial growth arrest during the first phase of infection The high proportion of bacteria that are still blocked in G1 phase at 6 h PI prompted us to investigate the growth and division status of B. abortus inside host cells. We first investigated the proportion of predivisional (Pd bacteria, constricting) at various times PI. Consistent with the invasive newborn hypothesis, we observed a low proportion of Pd displaying a cell constriction inside HeLa cells at 2, 4 and 6 h PI ( Fig. 4a ). Conversely, at 8, 10 and 12 h PI, the proportion of Pd bacteria increased to approximately reach the proportion of Pd bacteria detected in an exponential phase culture in rich medium. This data strongly suggests that growth is arrested during the first 6 h in HeLa cells. We therefore took advantage of the TRSE labelling to characterize the growth status of intracellular B. abortus at the single-cell level after 2, 4, 6, 8, 10 and 12 h PI ( Fig. 4b ). A majority of non-growing bacteria (totally TRSE labelled) were detectable at 2, 4 and 6 h PI (93%, 83% and 81% of cells, respectively), while the proportion of growing bacteria became increasingly predominant at 8, 10 and 12 h PI meaning that bacterial growth resumes between 6 and 8 h PI ( Fig. 4c ). These observations, well correlated with our observation of Pd cells proportions ( Fig. 4a ), confirmed the hypothesis of a general cell cycle arrest of B. abortus during the first phase of HeLa cells infection. 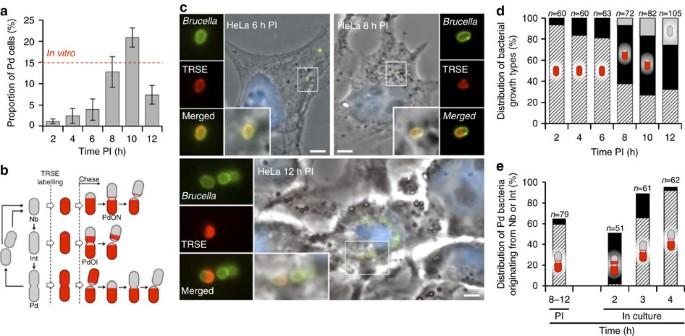Figure 4: Growth characterization ofB. abortusduring HeLa cells infection. (a) Proportion of Pd bacterial type at different times PI. The red dashed line represents the proportion of Pd bacteria detected in culture. Error bars represent s.d. The number of bacteria counted at 2, 4, 6, 8, 10 and 12 h PI is 357, 359, 372, 360, 376 and 385, respectively. One hundred and sixty-eight bacteria were counted in culture. (b) Schematic representation of the evolution of unipolarly growing cell types after a TRSE labelling (red areas). Nb stands for newborn, Int for intermediate and Pd for predivisional. PdON stands for predivisional originating from a newborn cell (weak TRSE labelling in the newly generated part) and PdOI for predivisional originating from an intermediate cell (partial TRSE labelling in the newly generated part). (c) Representative IF images of TRSE labelledB. abortusafter 6, 8 and 12 h of infection in HeLa cells. The bacteria were labelled in green. Scale bars, 1 μm. (d) Distribution of the three observed types of TRSE-labelled bacteria; completely labelled (hatched), partially labelled (black) and non-labelled (grey), at different times PI. Up to 6 h PI, the majority of bacteria show no sign of growth. The number of counted intracellular bacteria (n) is indicated for each time PI. (e) Growth resumption of TRSE-labelled bacteria at for 2, 3 or 4 h in culture or used for infection and observed after 8 to 12 h PI in HeLa cells. The proportion of PdON cells (dashed lines) or PdOI cells (black) was determined. After 8 to 12 h PI, the majority of the growing Pd cell types are originating from the Nb type (PdON). In culture, a majority of PdOI are observed before a complete generation time (that is, 3 h) suggesting that intermediate cells were predominant compared with newborns in culture. Figure 4: Growth characterization of B. abortus during HeLa cells infection. ( a ) Proportion of Pd bacterial type at different times PI. The red dashed line represents the proportion of Pd bacteria detected in culture. Error bars represent s.d. The number of bacteria counted at 2, 4, 6, 8, 10 and 12 h PI is 357, 359, 372, 360, 376 and 385, respectively. One hundred and sixty-eight bacteria were counted in culture. ( b ) Schematic representation of the evolution of unipolarly growing cell types after a TRSE labelling (red areas). Nb stands for newborn, Int for intermediate and Pd for predivisional. PdON stands for predivisional originating from a newborn cell (weak TRSE labelling in the newly generated part) and PdOI for predivisional originating from an intermediate cell (partial TRSE labelling in the newly generated part). ( c ) Representative IF images of TRSE labelled B. abortus after 6, 8 and 12 h of infection in HeLa cells. The bacteria were labelled in green. Scale bars, 1 μm. ( d ) Distribution of the three observed types of TRSE-labelled bacteria; completely labelled (hatched), partially labelled (black) and non-labelled (grey), at different times PI. Up to 6 h PI, the majority of bacteria show no sign of growth. The number of counted intracellular bacteria ( n ) is indicated for each time PI. ( e ) Growth resumption of TRSE-labelled bacteria at for 2, 3 or 4 h in culture or used for infection and observed after 8 to 12 h PI in HeLa cells. The proportion of PdON cells (dashed lines) or PdOI cells (black) was determined. After 8 to 12 h PI, the majority of the growing Pd cell types are originating from the Nb type (PdON). In culture, a majority of PdOI are observed before a complete generation time (that is, 3 h) suggesting that intermediate cells were predominant compared with newborns in culture. Full size image Furthermore, the majority of constricting bacteria at 8, 10 and 12 h PI displayed a TRSE labelling at only one of the two future daughter cells ( Fig. 4d ). This half-labelled predivisional cell type could only originate from the growth of a fully labelled newborn cell ( Fig. 4b , PdON), and not from Pd bacteria originating from Int cell type ( Fig. 4b , PdOI) that displayed more than half-TRSE labelling. Altogether, the intracellular growth characterization data are consistent with a model in which the newborn Brucella constitute the predominant invasive subpopulation. Bacterial cell cycle is resumed late in endosomal vacuoles As the transition between the non-proliferative (stable CFU) to the proliferative phase (increasing CFU) of the infection is correlated with the loss of Lamp-1 endosomal marker, we were expecting to observe the resumption of the B. abortus newborns cell cycle in the Lamp-1-negative compartments at 8 h PI. Indeed, during HeLa cell infections, a marked decrease of Lamp-1 labelling, indicating the exit from endosomal compartments, occurs between 8 and 12 h PI ( Fig. 5c ). In agreement with the absence of proliferation of B. abortus (that is, stable CFU) in Lamp-1-positive compartments in HeLa cells [3] , the majority (92%) of the newly generated daughter cells (not TRSE labelled) were only observed in Lamp-1-negative vacuoles ( Fig. 5a,b,e ). Unexpectedly, 63.3% of growing bacteria (that is, bacteria partially labelled with TRSE) were already observed in Lamp-1-associated compartments at 8 h PI ( Fig. 5a,e ). It is thus likely that bacterial growth starts in Lamp-1-positive compartments, but cell division is only completed when Lamp-1 labelling is lost. In order to confirm this interpretation, we used a virB deletion strain (Δ virB ) that is blocked in endosomes without proliferation [3] , predicting that this deletion strain could restart growing despite its unability to leave the Lamp-1 vacuoles. A TRSE-labelled Δ virB was still associated with the Lamp-1 marker at 8, 10 and 12 h PI, by contrast to the wild-type strain ( Fig. 5c ). At these times, a high proportion of growing bacteria (that is, partially labelled with TRSE) was detected but no newly generated bacterium was observed ( Fig. 5d ). These results indicate that even if B. abortus does not proliferate before leaving Lamp-1-positive compartments, 74 to 79% of the bacteria resume their growth within Lamp-1-associated vacuoles ( Fig. 5d ). We then tested if chromosomal replication was also reinitiated within a similar timing during the infection. We thus monitored oriI duplication (using a NoriI -targeted YFP-ParB pMT1 strain) and the labelling of Lamp-1 in HeLa cells at 6, 8 or 10 h PI ( Fig. 5g ). The proportions of bacteria having initiated their S phase were 26%, 46% and 54% at 6, 8 and 10 h PI, respectively ( Fig. 5f ). Moreover at 8 h PI, 73% of the bacteria displaying two NoriI foci were still associated with the Lamp-1 marker ( Fig. 5f ). Thus, similarly to growth, replication of the bacterial genome is reinitiated before leaving the Lamp-1-positive compartments, strongly suggesting a global resumption of B. abortus cell cycle within endosomal compartments. 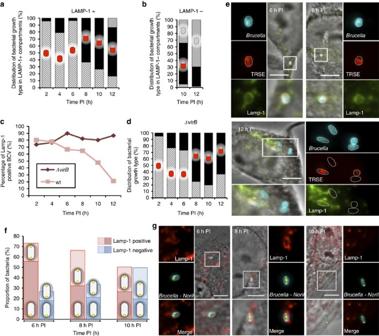Figure 5: Bacterial cell cycle resumes whileB. abortusis still associated with Lamp-1-positive compartments. (a) Distribution of the three observed types of TRSE-labelled bacteria; completely labelled (hatched), partially labelled (black) and unlabelled (grey), at different times PI in Lamp-1-positive compartments. At 8 h PI, a large proportion of bacteria residing in Lamp-1-positive compartments started to grow. Fourty-three to 103 bacteria are counted for each time PI. (b) Distribution of the bacterial growth types in Lamp-1-negative compartments at 10 and 12 h PI. The majority of newly generated bacteria (unlabelled by TRSE) are found in Lamp-1-negative compartments. (c) Proportion of Lamp-1-positiveBrucella-containing vacuoles (BCV) along the trafficking of the wild-type (wt) strain and the ΔvirBstrain. While the ΔvirBstrain-containing vacuoles retained Lamp-1 labelling, the wt strain lost Lamp-1 staining progressively, with a marked decrease at 10 and 12 h PI. (d) Distribution of the three observed types of TRSE-labelled bacteria in Lamp-1-positive compartments for the ΔvirBstrain. A majority of partially labelled bacteria are observed from 8 h PI, while no newly generated bacteria are observed at any time PI, in agreement with the previously reported absence of intracellular proliferation of thevirBmutant. 43 to 141 bacteria are counted for each time PI. (e) TRSE-labelledB. abortusstrain observed at 6, 8 and 12 h PI in HeLa cells labelled by anti-Lamp-1 staining. (f) Distribution of the foci number of YFP-labelledNoriIin Lamp-1 stained vacuoles in HeLa cells. In each type of vacuole (Lamp-1-positive or Lamp-1-negative), the proportion of bacteria with two foci of YFP-labelledNoriIis shown with a light colour. The proportion of bacteria displaying twoNoriIfoci increases in Lamp-1-positive compartments at 8 h PI and in Lamp-1-negative compartments at 10 h PI. The total number of counted bacteria was 223, 228 and 277 for 6, 8 and 10 h PI respectively. (g)B. abortusYFP-labelledNoriIstrain observed at 6, 8 and 10 h PI in HeLa cells labelled by anti-Lamp-1 staining. Scale bars represent 5 μm. Figure 5: Bacterial cell cycle resumes while B. abortus is still associated with Lamp-1-positive compartments. ( a ) Distribution of the three observed types of TRSE-labelled bacteria; completely labelled (hatched), partially labelled (black) and unlabelled (grey), at different times PI in Lamp-1-positive compartments. At 8 h PI, a large proportion of bacteria residing in Lamp-1-positive compartments started to grow. Fourty-three to 103 bacteria are counted for each time PI. ( b ) Distribution of the bacterial growth types in Lamp-1-negative compartments at 10 and 12 h PI. The majority of newly generated bacteria (unlabelled by TRSE) are found in Lamp-1-negative compartments. ( c ) Proportion of Lamp-1-positive Brucella -containing vacuoles (BCV) along the trafficking of the wild-type (wt) strain and the Δ virB strain. While the Δ virB strain-containing vacuoles retained Lamp-1 labelling, the wt strain lost Lamp-1 staining progressively, with a marked decrease at 10 and 12 h PI. ( d ) Distribution of the three observed types of TRSE-labelled bacteria in Lamp-1-positive compartments for the Δ virB strain. A majority of partially labelled bacteria are observed from 8 h PI, while no newly generated bacteria are observed at any time PI, in agreement with the previously reported absence of intracellular proliferation of the virB mutant. 43 to 141 bacteria are counted for each time PI. ( e ) TRSE-labelled B. abortus strain observed at 6, 8 and 12 h PI in HeLa cells labelled by anti-Lamp-1 staining. ( f ) Distribution of the foci number of YFP-labelled NoriI in Lamp-1 stained vacuoles in HeLa cells. In each type of vacuole (Lamp-1-positive or Lamp-1-negative), the proportion of bacteria with two foci of YFP-labelled NoriI is shown with a light colour. The proportion of bacteria displaying two NoriI foci increases in Lamp-1-positive compartments at 8 h PI and in Lamp-1-negative compartments at 10 h PI. The total number of counted bacteria was 223, 228 and 277 for 6, 8 and 10 h PI respectively. ( g ) B. abortus YFP-labelled NoriI strain observed at 6, 8 and 10 h PI in HeLa cells labelled by anti-Lamp-1 staining. Scale bars represent 5 μm. Full size image Invasive bacteria are mainly in G1 phase also in macrophages We tested the bacterial cell cycle arrest of B. abortus discovered in HeLa cells in professional phagocytes such as the RAW264.7 macrophages, which constitute another relevant cell type model for the study of infection by B. abortus [30] . Given that the replication initiation of chrI occurs before replication of chrII, the merodiploid mcherry-parB strain was chosen to investigate the genomic replication status of B. abortus in macrophages. We found that 72.9±3.1% ( n =495 of total bacteria) of the bacteria displayed only one mCherry-ParB ( oriI ) focus during the non-proliferative phase of infection (2 h PI) compared with the proliferative phase in which 45±2.2% of the bacteria ( n =1,381 of total bacteria) had only one mCherry-ParB focus ( Fig. 6a,b ). Similar to HeLa cells, one or two bacteria were also observed at 15 min PI with a very high proportion of B. abortus containing only one focus of NoriI region (77±1.6%, n =268 of total bacteria) ( Fig. 6c ). In addition, we found that the growth of B. abortus resumed between 4 and 6 h PI in macrophages and that the proportion of Pd cells starts to increase at 6 h PI ( Fig. 6d–f ). These results unexpectedly show that RAW264.7 macrophages infected by B. abortus are characterized from the onset of infection by the presence of only few bacteria per cell that are predominantly in the newborn status, similarly to non-professional phagocytes. 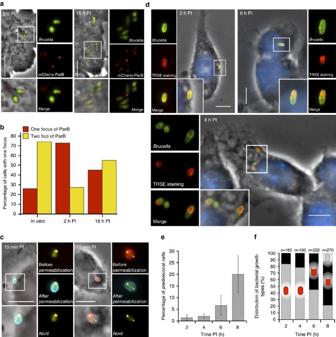Figure 6: G1 phase block and growth arrest ofB. abortusduring the non-proliferative phase of the infection in RAW264.7 macrophages. (a,b) Strain producing mCherry-ParB (red) and diffuse GFP (green) in RAW264.7 macrophages at 2 and 18 h PI. At 2 h PI, 72.9% of the bacteria display only one mCherry-ParB focus. (c)B. abortusYFP-labelledNoriIat 15 min PI after performing a dual labelling to discriminate between extracellular bacteria (red and cyan) from intracellular bacteria (cyan only). Only one or two intracellular bacteria were found per infected cell, these bacteria mainly displayed only one focus of YFP-labelledNoriI(77%). (d) TRSE-labelledB. abortusstrain observed at 2, 6 and 8 h PI in RAW264.7 macrophages. Scale bars in (a), (c) and (d) represent 5 μm. (e) Proportion of predivisional (Pd)B. abortusat 2, 4, 6 and 8 h PI (n=183, 190, 222 and 270, respectively). This proportion is higher at 8 h PI. Error bars represent s.d. (f) Distribution of the three observed types of TRSE-labelled bacteria; completely labelled (hatched), partially labelled (black) and non-labelled (grey), at different times PI in RAW264.7 macrophages. Up to 4 h PI, the majority of bacteria show no sign of growth. The number of counted intracellular bacteria (n) is indicated for each time PI. Figure 6: G1 phase block and growth arrest of B. abortus during the non-proliferative phase of the infection in RAW264.7 macrophages. ( a , b ) Strain producing mCherry-ParB (red) and diffuse GFP (green) in RAW264.7 macrophages at 2 and 18 h PI. At 2 h PI, 72.9% of the bacteria display only one mCherry-ParB focus. ( c ) B. abortus YFP-labelled NoriI at 15 min PI after performing a dual labelling to discriminate between extracellular bacteria (red and cyan) from intracellular bacteria (cyan only). Only one or two intracellular bacteria were found per infected cell, these bacteria mainly displayed only one focus of YFP-labelled NoriI (77%). ( d ) TRSE-labelled B. abortus strain observed at 2, 6 and 8 h PI in RAW264.7 macrophages. Scale bars in ( a ), ( c ) and ( d ) represent 5 μm. ( e ) Proportion of predivisional (Pd) B. abortus at 2, 4, 6 and 8 h PI ( n =183, 190, 222 and 270, respectively). This proportion is higher at 8 h PI. Error bars represent s.d. ( f ) Distribution of the three observed types of TRSE-labelled bacteria; completely labelled (hatched), partially labelled (black) and non-labelled (grey), at different times PI in RAW264.7 macrophages. Up to 4 h PI, the majority of bacteria show no sign of growth. The number of counted intracellular bacteria ( n ) is indicated for each time PI. Full size image Here, we report the characterization of the B. abortus cell cycle in culture and host cells with respect to growth and chromosome replication and segregation ( Fig. 7 ). We observed that the chrI centromere-binding protein mCherry-ParB displays a bipolar localization after initiation of chrI replication, suggesting that oriI is segregated similarly to the origin of replication of C. crescentus chromosome and V. cholerae chrI [19] , [23] . Concerning chrII, we showed that the duplicated YFP-RepB foci drift apart during cell growth without any visible sign of polar attachment. These observations provide for the first time the localization pattern of a protein member of the RepABC partitioning system ( Supplementary Fig. 5a,c and Supplementary Movie 1 ). In addition, the positions of NoriII and NterII regions in live bacterial cells showed no sign of chrII attachment in agreement with the conservation of plasmid-like features of chromids. These observations are consistent with the localization patterns of the origins of repABC -based replicons of Agrobacterium tumefaciens and Sinorhizobium meliloti using fluorescent in situ hybridization in fixed cells [14] . Moreover, our fluorescent reporters also showed that the replication of chrII is initiated after origin duplication of chrI suggesting the presence of an unknown mechanism coordinating these events in time. Interestingly, it was recently reported that a specific site located in chrI was able to enhance chrII replication in V. cholerae [31] . The analysis of the foci number of both terminators also suggests that the segregation of terII occurs well before cell septation, while terI segregation was observed in constricting cells. These two observations are similar to those reported for V. cholerae chromosomes [19] , [27] , [29] , [32] . However, the chrII origin in B. abortus displays a looser localization pattern (before and after duplication) compared with the V. cholerae oriII . This could result from a different molecular mechanism of segregation for the RepAB system, which remains to be investigated ( Fig. 2a–d ). 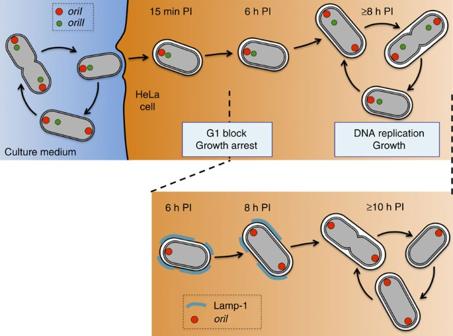Figure 7: Model of theB. abortuscell cycle outside and inside host cells. During theB. abortuscell cycle, replication of chrI is initiated before chrII. NewbornB. abortus(in G1) are proposed to be the predominantly invasive cell type for host cells. Indeed, between 15 min and 6 h PI, that is, the non-proliferative stage of the infection, bacteria are found as non-growing cells blocked before the replication initiation of the two chromosomes. Growth and chromosomal replication are reiniated in Lamp-1-positive compartments at 8 h PI (lower panel), and cell division is completed in Lamp-1-negative compartments, where bacteria subsequently proliferate. Figure 7: Model of the B. abortus cell cycle outside and inside host cells. During the B. abortus cell cycle, replication of chrI is initiated before chrII. Newborn B. abortus (in G1) are proposed to be the predominantly invasive cell type for host cells. Indeed, between 15 min and 6 h PI, that is, the non-proliferative stage of the infection, bacteria are found as non-growing cells blocked before the replication initiation of the two chromosomes. Growth and chromosomal replication are reiniated in Lamp-1-positive compartments at 8 h PI (lower panel), and cell division is completed in Lamp-1-negative compartments, where bacteria subsequently proliferate. Full size image Importantly, we also report the predominance of a B. abortus cell type during the non-proliferative phase of HeLa cells infection corresponding to the newborn (G1) stage of the bacterial cell cycle, which is present in minority in culture conditions. Indeed, during this phase of infection, the majority of intracellular bacteria are characterized by (i) a striking growth arrest shown by TRSE labelling and (ii) the unreplicated status of both chromosomes (G1 block) indicated by single foci of the origin markers mCherry-ParB and YFP-RepB ( Fig. 7 ). This population regroups the majority of the intracellular B. abortus right after entry into the host cell (15 min PI), demonstrating that they must have entered the HeLa cells in this infectious newborn state. Hence, we named this subpopulation ‘infectious newborn’. In addition, a similar conclusion is reached after the observation of essentially newborn bacteria during the non-proliferative phase of infection in macrophages, showing that the predominance of the infectious newborn subpopulation is not just limited to non-professional phagocytes like HeLa cells. This is surprising because macrophages were traditionally thought to actively uptake large numbers of bacteria and then quickly kill a vast majority of them. Thus, the specific internalization of a bacterial subpopulation suggests that B. abortus controls the process, instead of being ‘passively’ phagocytosed. It would be interesting to test different types of macrophages (primary cultures and other cell lines) to further investigate the preferential entry of newborns. How this subpopulation is specifically competent for internalization is currently unknown but could be linked to the presence of polar adhesins mediating contact between bacteria and host cells [33] , [34] . In addition, our data strongly suggest that intracellular bacteria resume growth and genome replication before losing the Lamp-1 marker, in a VirB-independent manner. Interestingly, B. abortus proliferates in Lamp-1-positive compartments in human extravillous trophoblasts [35] . The ability to resume the bacterial cell cycle in endosomal compartments could therefore be a general feature, independent of the maturation of the vacuole into an ER-like compartment. On entry, the bacteria are exposed to an environment deprived of nutrients [36] , which would explain the strong attenuation of mutants unable to efficiently adapt to starvation [37] . Starvation is known to trigger a growth arrest that will in turn lead to an endogenous accumulation of oxidative DNA damages [38] . Other detrimental stresses like acidic pH or reactive oxygen species-related damages encountered during the non-proliferative phase of infection could also promote a cell cycle arrest [36] . It is thus likely that an inhibition of growth and repression of DNA replication have been selected to adapt to starvation until bacteria reach an environment permissive for their proliferation. In fact, we speculate that DNA replication could be detrimental if occurring under harsh conditions encountered within the host cell, such as an increasing amount of reactive oxygen species [39] . Hence, at the evolutionary level, the specific entry of newborns present in a mixed population could have been selected because these cells do not undergo DNA replication, as part of the arsenal allowing Brucella to survive in harmful environments. Since Salmonella , Legionella , Chlamydia and Francisella cellular infections also display a lag phase [1] , it would be worth investigating whether a particular control of their cell cycle also occurs before resuming intracellular proliferation. Recently, a subpopulation of intramacrophagic non-replicating Salmonella was proposed to contribute to the persistence of these bacteria during infection [40] . In the light of our discovery, it would therefore be fundamental to determine the stage of the bacterial cell cycle in which the persister populations of intracellular pathogens are blocked. Regarding brucellosis, it would also be interesting to investigate the ability of Brucellae to generate persisters, since Brucella infection leads to a chronic disease. Finally, it is also tempting to relate the growth arrest and G1 block of intracellular B. abortus to the C. crescentus differentiation model, in which each division generates a swarmer cell type blocked before the S phase as long as starvation is sensed [41] . This suggests that an environment-dependent G1 arrest could be a very ancient trait among alphaproteobacteria. We propose that this trait could be shared by other bacterial taxons for adaptation during the colonization of new environments where nutrients availability and the presence of toxic compounds can sharply fluctuate. Bacterial strains All Brucella strains used in this study were routinely cultivated in 2YT rich medium (1% yeast extract, 1.6% peptone, 0.5% NaCl). All E. coli strains were grown in Luria-Bertani broth, except for strain STBL2 which was grown in M9 medium. Antibiotics were used at the following concentrations when appropriate: nalidixic acid, 25 μg ml −1 ; kanamycin, 15 (STBL2), 20 or 50 μg ml −1 ; chloramphenicol, 20 μg ml −1 ; ampicillin, 100 μg ml −1 ; gentamicin, 15 (STBL2) or 50 μg ml −1 ; rifampicin 20 μg ml −1 . Oxytetracycline inducer was used at 12 μg ml −1 . Plasmids were mobilized from E. coli strain S17-1 (ref. 42 ) to B. abortus 544 Nal R . Strains constructions are described in Supplementary Methods , bacterial strains are listed in Supplementary Table 1 , plasmids are indicated in Supplementary Table 2 and primer sequences are provided in Supplementary Table 3 . TRSE labelling Cultures of B. abortus were centrifugated at 2,500 g for 2 min and washed thrice in phosphate-buffered saline (PBS) at room temperature (RT). Cell pellets were resuspended with Texas Red Succinimidyl Ester (Invitrogen) in PBS at a concentration of 1 μg ml −1 and incubated for 15 min in the dark [12] . Then, the bacteria were washed twice in PBS and once in Dulbecco’s Modified Eagle’s Medium (DMEM) to obtain the inoculum used for the infection. For growth assays, the bacteria were resuspended in fresh 2YT medium. HeLa cell and RAW264.7 macrophages cultures and infections HeLa cells (from the Centre d'Immunologie de Marseille-Luminy, Marseille, France) were cultured at 37 °C in a 5% CO 2 atmosphere in DMEM (Invitrogen) supplemented with 10% fetal bovine serum (Gibco), 0.1 g l −1 non-essential amino acids (Invitrogen) and 0.1 g l −1 sodium pyruvate. RAW264.7 macrophages (from ATCC) were cultured at 37 °C in a 5% CO 2 atmosphere in DMEM (Invitrogen) supplemented with 10% fetal bovine serum (Gibco), 4.5 g l −1 glucose, 1.5 g l −1 NaHCO 3 and 4 mM glutamine. Cultures of Brucella were prepared in DMEM at a multiplicity of infection of 300 or 1,000 bacteria per cell for HeLa cells infection and at a multiplicity of infection of 50 for RAW264.7 macrophages infection. Bacteria were centrifuged at 400 g for 10 min at 4 °C and then incubated for 1 h at 37 °C with 5% CO 2 atmosphere. Cells were washed twice with fresh medium and then incubated in medium supplemented with 50 μg ml −1 gentamicin to kill extracellular bacteria. Immunolabeling of infected hosts cells Cells were washed three times with PBS, then fixed in 2% paraformaldehyde (PFA), pH 7.4, at RT for 20 min, and permeabilized with Triton-X-100 (Prolabo) 0.1%, during 10 min. Primary and secondary antibodies were diluted in PBS containing 0.1% Triton and 3% bovine serum albumin (BSA, Sigma Aldrich). The immunodetection of intracellular Brucella was made with a A76-12G12 monoclonal antibody [43] (hybridoma culture supernatant not diluted) followed by a goat anti-mouse secondary antibodies coupled to Alexa 488 or Texas red diluted 500 times (Sigma Aldrich). The 4′,6-diamidino-2-phenylindole (1 μg ml −1 ) staining was used to detect nuclei. The coverslips were washed three times with PBS, then once with dd H 2 O and mounted with Mowiol (Sigma). For living infected HeLa cells with sXDB021 observations, cells were infected as indicated above. At the time of the observation, cells were washed three times with PBS and the coverslips were directly flipped on agarose pads. Before the observation, pads were sealed and successively treated with incidine 2% for 5 min and ethanol 70% for 5 min for decontamination. Internalization assay At 15 min PI, infected HeLa cells were fixed in 2% PFA, pH 7.4, at RT for 20 min. The immunodetection of extracellular bacteria was performed for 1 h with a homemade rabbit serum against Brucella diluted 2,000 times in PBS with 3% BSA. After permeabilization with 0.1% Triton-X-100 (Prolabo) for 10 min, the coverslips were incubated for 1 h at RT with anti-lipopolysaccharide A76-12G12 monoclonal antibody [43] (undiluted), washed three times with PBS and incubated with secondary antibodies solution (each diluted 500 times) containing a donkey anti-rabbit coupled to Alexa 488 (Sigma Aldrich), a goat anti-mouse coupled to Texas red (Sigma Aldrich), in PBS with 3% BSA 3% and 0.1% Triton-X-100, for 1 h at RT. The coverslips were washed three times with PBS, then once with water and mounted with Mowiol (Sigma Aldrich). The homemade anti- Brucella serum was obtained by immunizing two rabbits with fixed Brucella melitensis 16 M or B. abortus 544 alternatively; thus, each rabbit generated an antiserum for both bacterial strains. Briefly, bacterial cultures (1 ml) were fixed with 2% PFA, washed with PBS and mixed with complete Freund adjuvant for intradermic injections at day 1. The injections were repeated with incomplete Freund adjuvant at days 28 and 56. Afterwards, the rabbits were injected every 3 months for a period of 9 months. Serum was collected every month after day 56. MicrobeTracker and matlab analyses Cell meshes were obtained using the open source, Matlab-based MicrobeTracker software [44] . Foci detections were automatically obtained from the SpotFinderZ tool of MicrobeTracker followed by manual verification with SpotFinderM. Further quantitative analyses from cell meshes were performed with Matlab software (The MathWorks Inc., Natick, MA). Demographs were obtained using scripts derived from [45] . Orientations of the meshes were performed as described in ref. 46 . New pole labelling IfoP-YFP fluorescent signal was used for the orientation of XDB005. Old-pole labelling PdhS-mCherry fluorescent signal or TRSE labelling were used for meshes orientation of XDB009 and XDB016 strains. New pole PopZ-mCherry fluorescent signal was used for meshes orientation of XDB012 strain. Fluorescent signal from mCherry-ParB fusion was used for orientation of XDB019 strain. Coldoplot script was used for generating Supplementary Figs 2e and 5b (Copyright (c) 2010, Per Sundqvist. All rights reserved). Microscopy Brucella strains and infected HeLa cells were observed with a Nikon 80i (objective phase contrast × 100, plan Apo) connected to a Hamamatsu ORCA-ER camera. For the observation of bacteria, 1.5 μl of an exponential phase culture was dropped on agarose pad (solution of 1% agarose in PBS) and sealed with VALAP (1/3 of vaseline, 1/3 of lanoline and 1/3 of paraffin wax). Time-lapse experiments with B. abortus strains were performed from cultures in exponential phase in liquid Plommet–erythritol containing K 2 HPO 4 (0.92 g l −1 ), KH 2 PO 4 (3 g l −1 ), Na 2 S 2 O 3 (0.1 g l −1 ), NaCl (5 g l −1 ), Nicotinate (0.2 g l −1 ), Thiamine (0.2 g l −1 ), (NH 4 ) 2 SO 4 (0.5 g l −1 ), Pantothenate (0.07 g l −1 ), Erythritol (2 g l −1 ), MgSO 4 ·7H 2 O (10 g l −1 ), MnSO 4 (1.1 g l −1 ), FeSO 4 ·7H 2 O (1 g l −1 ) and Biotine (1 g l −1 ). Cultures were spread on a sealed Plommet–erythritol agarose 1% pad. Images were automatically taken every 20 min at 32 °C with NIS-Element software (Nikon). Imaging of E. coli strains was performed using either a Nikon Eclipse 80i microscope equipped with a Hamamatsu Orca II-ER camera ( × 100 differential interference contrast or phase-contrast objectives, optivar × 1.5 when appropriate) or a Nikon Eclipse Ti-U with a Hamamatsu Orca-ER LCD camera ( × 100 phase-contrast objective). Images were processed with Metamorph software (Molecular Devices, Sunnyvale, CA). Flow cytometry analysis Flow cytometry analyses were performed on XDB001, XDB003, XDB004, XDB011, XDB018 and XDB019 strains. Cultures in exponential phase were treated for 6 h with rifampicin (20 μg ml −1 ) in the same culture medium. One ml of each culture was collected and mixed with 9 ml of ice-cold 77% ethanol for inactivation and permeabilization for at least 4 h. Two ml of the fixed cells were washed two times in 2 ml of flow cytometry staining buffer (10 mM of Tris, pH 7.2, 1 mM of EDTA, 50 mM of sodium citrate and 0.01% of Triton-X-100) supplemented with 0.1 mg ml −1 of RNAse A for 30 min at RT, washed again and resuspended in 1 ml of flow cytometry staining buffer supplemented with 0.5 μM of Sytox Green (Invitrogen). For each flow cytometry analysis, fluorescence corresponding to DNA content in a population of 250,000 cells was measured with a FACScalibur using CellQuest software (Becton Dickinson) with excitation at 495 nm and emission at 519 nm. How to cite this article: Deghelt, M. et al. G1-arrested newborn cells are the predominant infectious form of the pathogen Brucella abortus . Nat. Commun. 5:4366 doi: 10.1038/ncomms5366 (2014).